Merging of metal nanoparticles driven by selective wettability of silver nanostructures The welding and sintering of nanomaterials is relevant, for example, to form electrical contacts between metallic particles in printed electronic devices. Usually the welding of nanoparticles is achieved at high temperatures. Here we find that merging of two different metals, silver and gold nanoparticles, occurs on contact at room temperature. The merging process was investigated by experimental and molecular dynamics simulations. We discovered that the merging of these particles is driven by selective wettability of silver nanoparticles, independent of their size and shape (spheres or rods); silver behaves as a soft matter, whereas gold as a hard surface being wetted and retaining its original morphology. During that process, the silver atoms move towards the surface of the Au nanoparticles and wrap the Au nanoparticles in a pulling up-like process, leading to the wetting of Au nanoparticles. Welding and sintering of various metal nanoparticles (NPs) were intensively investigated during the last decade [1] , [2] , [3] , [4] , [5] , [6] . The main driving force for that research is the challenge to form electrical contacts between nanoscale metal particles in nanoelectronic devices and nanoelectromechanical systems, particularly in printed electronics [7] , [8] . Already in 1909, Pawlow [9] predicted a decrease in the melting point of such metallic NPs, and Buffat and Borel [10] demonstrated it on gold. A decrease in melting point was attributed to the diffusion of metal atoms at the surface of the metal NPs, which increases with the rise in temperature. Later on, a dependence of the melting temperature on a size of a gold NP was studied by Cleveland et al . [11] and Dick et al . [12] Recently, a coalescence of either silver or gold NPs was shown to take place even at room temperature [13] , [14] . The process, which is triggered by the removal or delocalization of the capping molecules at the surface of the NPs, takes place spontaneously once two NPs come into contact due to atom diffusion at the surface. Other techniques, including Ar plasma [15] , [16] , were shown to lead to the same phenomena—room-temperature coalescence of the metallic NPs—simply by decomposing the capping molecules, which prevent contact between the NPs. These findings led to the suggestion that interaction of nanodimensional metal particles at low temperatures resembles coalescence behaviour of soft matter [13] , [17] and high-temperature sintering of ceramics [18] . Still, all these reports focused on homogeneous NP systems in which interaction of NPs of the same elemental composition was observed [19] , [20] , [21] , [22] . In the present work, we studied experimentally by transmission electron microscopy (TEM) and theoretically via molecular dynamics simulation an interparticle interaction in heterogeneous system containing NPs of differing metals, Au and Ag, with dissimilar morphology (sphere- and rod-type NPs). It was found that such systems present a unique, wetting-like phenomenon; on contact of two dissimilar NPs, Ag behaves as a soft matter that wets an Au particle, whereas the Au remains almost intact. The wetting process results in merging of the particles, which then share a stable atomic interface without detectable alloying ( Supplementary Fig. S1 ). Experimental results of Ag wetting on Au surfaces The above phenomenon was observed while depositing together Ag and Au nanomaterials by mixing two aqueous dispersions and drying on TEM grid. To increase the probability of contact between Au and Ag NPs, we employed different shapes, Ag nanospheres or nanorods (NRs) mixed with Au NRs or nanoshperes, respectively. 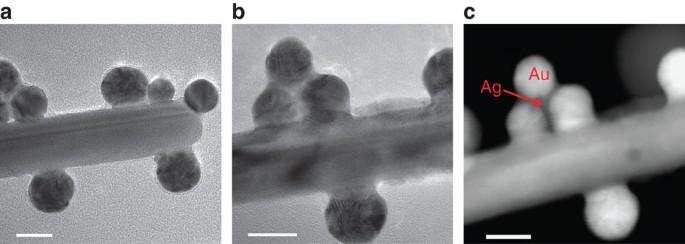Figure 1: Electron microscopy characterization of Au NPs on Ag NR. Bright-field TEM (a,b) and high-angle annular dark-field STEM (c) images of gold NPs contacting a silver NR; all scale bars, 20 nm. It is clearly seen that the gold NPs do not change, whereas the silver NR ‘climbs’ to wet the gold spheres. Figure 1 shows the result of the contact between Au NPs and an Ag NR. Initially ( Fig. 1a ), the projected view of the outer facet of the Ag NR looks flat and after 10 min it became curved (see changes between snapshots a and b), whereas the Au NPs remained almost unchanged ( Supplementary Fig. S2 ). Furthermore, as shown in the upper part of Fig. 1b , where a group of three Au NPs are present on the Ag NR, we observed a ‘soaking-like’ process in which the gap between the three Au NPs is filled. The energy dispersive X-Ray spectroscopy image presented in Fig. 1c reveals that the space between the three Au NPs was filled with Ag ( Supplementary Fig. S3 ). A similar phenomenon is observed at the bottom of Fig. 1b,c , in which the Ag climbs towards the Au NPs and forms a cup-like Ag ‘carrying’ an Au NP (the bright domains in Fig. 1c with a stronger signal represent Au, whereas darker grey domains with lower signal level represent Ag, Supplementary Fig. S3 ). Figure 1: Electron microscopy characterization of Au NPs on Ag NR. Bright-field TEM ( a , b ) and high-angle annular dark-field STEM ( c ) images of gold NPs contacting a silver NR; all scale bars, 20 nm. It is clearly seen that the gold NPs do not change, whereas the silver NR ‘climbs’ to wet the gold spheres. Full size image It should be emphasized that these results are in contradiction with the well-known Ostwald ripening phenomenon. A small sphere is expected to be soaked by the large rod, while here we observe how the small, spherical Au NP exhibited exceptional stability on contact with the large Ag NR. Therefore, we may conclude from the TEM and scanning TEM (STEM) data that the Ag NR behaves as a soft matter, whereas the Au NP behaves as a solid body. The soft-like behaviour of Ag is even more striking while observing the reverse case, in which an Ag NP contacts an Au NR. As presented in Fig. 2 , such a contact leads not only to the merging of the Ag with the Au but to a wetting-like phenomenon of the Ag over the Au. In this case (Ag NP over an Au NR), it is clearly seen how the deformation of the Ag NP proceeds until its shape was totally changed, while the Au retained its rod morphology. At the beginning, the Ag NP was attached to the Au NR, then the silver particle spreads over the surface of the Au NR until complete merging of the Ag and Au occurred. 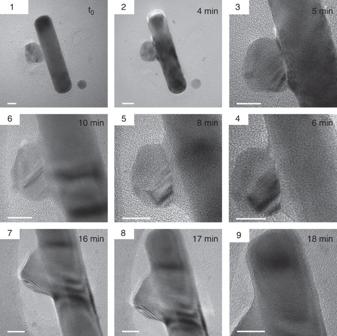Figure 2: Electron microscopy characterization of Ag NP on Au NR. HR-TEM images showing the merging of silver NP with the gold nanorod, all scale bars 10nm. Snapshots of interaction between a gold nanorod and a silver NP taken in TEM. The time stamp is indicated on the upper right corner of each image. Figure 2: Electron microscopy characterization of Ag NP on Au NR. HR-TEM images showing the merging of silver NP with the gold nanorod, all scale bars 10nm. Snapshots of interaction between a gold nanorod and a silver NP taken in TEM. The time stamp is indicated on the upper right corner of each image. Full size image The wetting of an Ag NP over an Au NR is even better observed in the STEM images presented in Fig. 3 for two Ag NPs merged on the two edges of an Au NR. Elemental mapping of the Ag and Au over that marked area confirms the selective wetting of the Ag over the Au, while the Au NR totally retains its morphology. 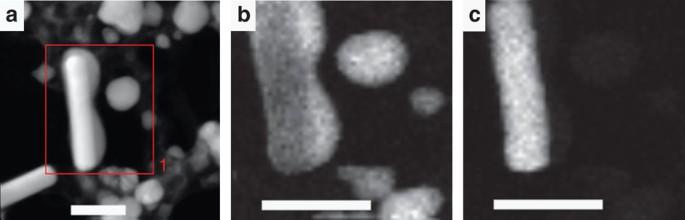Figure 3: Elemental mapping of merged particles. STEM images (a) and elemental mapping of Ag (b) and Au (c); all scale bars, 50 nm. Figure 3: Elemental mapping of merged particles. STEM images ( a ) and elemental mapping of Ag ( b ) and Au ( c ); all scale bars, 50 nm. Full size image Molecular dynamics simulations of Ag–Au interfaces To understand this unique phenomenon, molecular dynamics simulation was carried out to track the detailed motion of the contact of Ag and Au for both cases, that is, an Au NP over an Ag NR and an Ag NP over an Au NR. As noble metal NPs acquire a polyhedron morphology at nanoscale [23] , we started with the Au and Ag NPs in the form of polyhedral. To verify the general concept, we studied various scenarios for particles with different cleavage options with different facets, different shapes including both decahedron and icosahedron, and different sizes. The NRs studied were with different facets and surfaces with different diameters (10 nm length). We found that the wetting-driven merging phenomena observed in this work hold for all the simulations and is not dependent on particle size (similar to the experimental observations for a variety of particle sizes, both NR and NP, independent of their size). Here we present the simulation results with NPs and NRs bound mainly with {111} facets (additional simulation scenarios are presented in the Supplementary Fig. S4 ). It can be seen that in the case of Au NP over an Ag NR ( Fig. 4a ), once the Au NP came into contact with the Ag NR (at 300 K) the Au NP did not wet the Ag NR. The silver atoms moved towards the surface of the Au NP, started wrapping the Au NP in a pulling up-like process, leading to the wetting on Au NP. This unexpected wetting phenomenon, in which Ag atoms wrap the Au particle in a pulling up-like manner, is due to two important factors. First, the better structural adaptive characteristics of Ag favours the disruptive deformation in the Ag. Second, the integrity of the Au particle is very well preserved, especially at room temperature. Consequently, Ag atoms are actively diffused upwards along the contact between Ag NR and Au NP, which is well presented by analysing the radial distribution function of Ag atom diffused in the vicinity of the contact ( Supplementary Fig. S5 ). 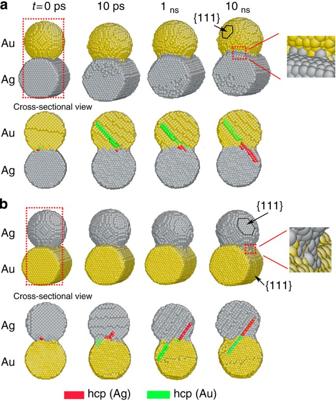Figure 4: Molecular dynamics simulation of merging particles. Molecular dynamics simulations of an Au NP over an Ag NR (a) and an Ag NP over an Au NR (b) at room temperature. The intriguing wetting phenomenon occurs, in which Ag atoms wrap the Au NR in a pulling up-like manner as presented ina. The Ag cluster gradually wets and merges the surface of Au NR at room temperature inb. Partial dislocations and face-centred cubic/hexagonal close-packed stacking faults near the junction between NPs and NR are energetically favourable to align up across the junction, which can facilitate the merging process. Au and Ag atoms are represented by yellow and grey coloured balls, respectively. Figure 4: Molecular dynamics simulation of merging particles. Molecular dynamics simulations of an Au NP over an Ag NR ( a ) and an Ag NP over an Au NR ( b ) at room temperature. The intriguing wetting phenomenon occurs, in which Ag atoms wrap the Au NR in a pulling up-like manner as presented in a . The Ag cluster gradually wets and merges the surface of Au NR at room temperature in b . Partial dislocations and face-centred cubic/hexagonal close-packed stacking faults near the junction between NPs and NR are energetically favourable to align up across the junction, which can facilitate the merging process. Au and Ag atoms are represented by yellow and grey coloured balls, respectively. Full size image In the reverse case ( Fig. 4b ), the Ag NP came into contact with the Au NR. The atomic diffusion on the metallic surface can be thermally activated at room temperature. Moreover, the Ag atoms on the surface were more energetic than those in the interior. Hence, Ag atoms in the peripheral surface of the contact were more diffusive with Au atoms nearby. The structurally adaptive potential of Ag atoms has also been reported previously for the growth of metastable Ag icosahedra [23] and cold welding of Ag nanowires with applied low pressure [23] , [24] . The whole process (in both cases) is realized by the movement of Ag atoms over the Au surface, which is actually a wetting phenomenon, that occurs at room temperature, much below the melting points of bulk Ag and Au (1,234.9 and 1,337.3 K, respectively). For the contact made of Ag NPs on Au NRs, the average angle is 145° ( Supplementary Fig. S5 ). For both Au NP on Ag NR and Ag NP on Au NR, beyond the intrinsic face-centred cubic stacking pattern in the Ag and Au, evolution of intrinsic local defects such as stacking faults and partial dislocations are presented during the merging ( Supplementary Fig. S6 ). Partial dislocations and stacking faults near the junction between NPs and NRs are energetically favourable to align up across the junction, which can facilitate the merging, as clearly shown after 20 ns for both cases. Interestingly, as shown in Fig. 4b , after 10 ns the polyhedron structure transforms into a less-ordered structure. The simulation results are in agreement with the experimental results and mean that Ag is a ‘softer metal’ than Au and, therefore, is capable of wetting the Au surface. As reported, Au and Ag have different surface tensions above their melting point, 0.89 and 1.13 N m −2 (at 1,381 K), and usually as the liquid with the lower surface tension will wet the one with the higher surface tension, a similar wetting behaviour at the molten state would occur [25] . Note that the melting temperature of a material is proportional to its cohesive energy, according to the Lindemann criterion [26] . The cohesive energy of Ag is 2.95 eV per atom, which is much weaker as compared with that of Au, that is, 3.81 eV per atom. As more prominent melting point reduction is anticipated for Ag nanostructures [27] , the liquid-like state is more accessible near the surfaces of Ag NPs. It is energetically favourable to break an Ag–Ag bond and to form an Ag–Au bond to gain 0.36 eV per pair. Therefore, it can be concluded that the pulling up-like process is the manifestation of the intrinsic characteristics of Ag NPs rather than the commonly encountered anisotropic diffusion and growth mode facilitated by the Ehrlich–Schwoebel barrier [28] , [29] . We emphasize that the proposed mechanism of wetting should have limitations, as we studied only two specific metals, Au and Ag. The effect of the nature of the two materials on the wetting-driven welding requires further study with other pairs of nanomaterials. The exotic, selective wetting and merging dynamics first observed in this work, and supported by dynamic simulations, make one important step forward in heuristic understanding of the complex interplay between thermodynamics and interfacial microstructures. Synthesis of sphere-like Au NPs Au NPs were synthesized by reducing HAuCl 4 with trisodium citrate. Ten milligrams of HAuCl 4 ·3H 2 O was dissolved in 100 ml of triple distilled water. Next, 2.5 ml of 1 wt% trisodium citrate was added and the mixture was heated to 95 °C in a hot bath while stirring. After 20 min of incubation, the solution turned red and the dispersion was cooled in an ice bath. Synthesis of sphere-like Ag NPs Ag NPs were synthesized by reducing AgNO 3 with trisodium citrate. AgNO 3 (1.8 ml of 1 wt%) was added to 100 ml of triple distilled water. Next, 4 ml of 1 wt% trisodium citrate was added and the mixture was heated to 95 °C in a hot bath while stirring. Synthesis of Ag NRs Ag NRs were synthesized by reducing AgNO 3 with trisodium citrate. AgNO 3 (1.8 ml of 1 wt%) was added to 100 ml of triple distilled water. Next, 4 ml of 1 wt% trisodium citrate was added and the mixture was heated to 95 °C in a hot bath while stirring. After 15 min of incubation, 0.5 ml 1 wt% of AgNO 3 was added. The addition of 0.5 ml of 1 wt% AgNO 3 was repeated six times (10 min between each addition), then the dispersion was cooled in an ice bath. The Au NRs, 25 nm in diameter and 113 nm in length (model number A12-25-850), were purchased from Nanopartz, USA. These NRs are capped by cetyl trimethyl ammonium bromide. Preparation of a mixture of Au and Ag NPs Equal amounts of both dispersions (either Ag NRs with Au NPs or Ag NPs with Au NRs) were mixed and treated with a mechanical stirrer for ~1 min. Next, 3.5 μl drop of the resulting dispersion was deposited on a carbon-coated 400-mesh copper TEM grid, which was subsequently dried in a vacuum chamber (~10 −2 Torr) for 2 min. Characterization methods STEM Tecnai F20 G 2 (FEI) was used for the observation and characterization of particles’ interaction in TEM, high-resolution TEM, STEM modes and energy dispersive X-Ray spectroscopy characterizations. Simulations methodology Molecular dynamics simulation was performed with the Verlet algorithm, where all the atoms were coupled with a Nose–Hoover thermostat [30] at a constant temperature of 300 K under the canonical ensemble with NVT (fixed number of atoms, constant volume, constant temperature). The time integration step for the equation of motion of the simulation is 0.2 fs. The embedded atom method [31] is implemented to describe the interatomic potential of Ag and Au atoms, which leads to the excellent description of the many-electron nature of chemical bonding and phonon dispersion in both Ag and Au materials as compared with experimental measurements [32] , [33] . Furthermore, this alloy-based embedded atom model (EAM) potential can reproduce experimental data with good agreement on lattice parameter, bulk modulus, cohesive energy, elastic constants, sublimation energies and heats of solution (for more justification regarding the EAM potential, see Supplementary Fig. S7 ). The equation of state derived directly from the potential parameters nicely demonstrate the higher cohesive energy, larger surface tension and larger bulk modulus of Au bulk state as compared with Ag. The EAM potential used here also enabled Pereira and da Silva [24] to perform simulations of welding of gold and silver nanowires with diameters of 4.3 nm by applying pressure. In our work, no pressure is applied in simulating the wetting-driven welding process between NPs and NRs [31] , [34] . How to cite this article: Grouchko, M. et al . Merging of metal nanoparticles driven by selective wettability of silver nanostructures. Nat. Commun. 5:2994 doi: 10.1038/ncomms3994 (2014).